Two-dimensional structure from random multiparticle X-ray scattering images using cross-correlations Knowledge of the structure of biological macromolecules, especially in their native environment, is crucial because of the close structure–function relationship. X-ray small-angle scattering is used to determine the shape of particles in solution, but the achievable resolution is limited owing to averaging over particle orientations. In 1977, Kam proposed to obtain additional structural information from the cross-correlation of the scattering intensities. Here we develop the method in two dimensions, and give a procedure by which the single-particle diffraction pattern is extracted in a model-independent way from the correlations. We demonstrate its application to a large set of synchrotron X-ray scattering images on ensembles of identical, randomly oriented particles of 350 or 200 nm in size. The obtained 15 nm resolution in the reconstructed shape is independent of the number of scatterers. The results are discussed in view of proposed ‘snapshot’ scattering by molecules in the liquid phase at X-ray free-electron lasers. The majority of macromolecular structures currently available at atomic resolution has resulted from X-ray cryo-crystallography at synchrotrons, which requires crystals larger than a few micrometres to avoid excessive radiation damage [1] . Three-dimensional (3D) molecular shapes may also be extracted from solution small-angle X-ray scattering (SAXS) [2] , [3] , whereby the few nanometers limit in the resolution [4] , [5] is owing to the fact that only the isotropic component of the single-particle scattering intensity is accessible. The advent of X-ray free-electron lasers (XFELs) [6] is stimulating the emergence of new imaging methodologies [7] , [8] . Among these is serial crystallography on easier-to-grow submicrometer crystals, in the ‘diffract-and-destroy’ mode, which was recently demonstrated to provide near-atomic resolution [9] . However, accessing structural information on non-crystalline and non-oriented samples beyond the capabilities of SAXS remains challenging. Snapshot diffraction from single particles has been considered by several groups [10] , [11] , [12] , motivated by the high-intensity of the fs-duration XFEL pulses. But despite the enormous increase in peak brilliance, a typical XFEL single-shot diffraction image of an isolated biomolecule is predicted to yield much less than one photon per coherent pixel at the relevant resolution, requiring sophisticated statistical and computational methods for establishing the model of the 3D diffraction intensity, which is in best agreement with the noisy experimental data [10] , [11] . A remarkable alternative, which exploits the same features of XFEL radiation, is the method proposed already in 1977 by Kam [13] , who suggested evaluating the cross-correlations (CCs) of the scattered intensity from identical particles in solution. These correlations are sensitive to angular fluctuations, which are averaged out in the traditional SAXS analysis. The disadvantage of the CC method, that the single-particle diffraction pattern must be derived indirectly, is largely compensated by the fact that multiparticle scattering is implicitly allowed, that experimental complications such as background scattering and non-uniform beam profile are easily accounted for, and, most importantly, that dealing with the large number of scattering images necessary to counteract the low photon count rates is absolutely straightforward. For our demonstration experiment at a synchrotron source, the reduced X-ray beam fluence was made up for by using strongly scattering nanostructures, and by immobilizing them to permit arbitrarily long acquisition. Liquid-state behaviour was mimicked by illuminating different random configurations of particles. Reducing the number of effective dimensions in the problem from three to two simplified both sample preparation and CC data analysis. Such an experiment was recently proposed [14] , [15] and realized with nanocylinders [16] . However, the reconstructed structure is obscured by a prominent ball-shaped feature, and the claimed resolution is of the order of the small cylinder dimension, both of which limit the image quality. We report here 2D structural determinations of gold nanoparticles exhibiting threefold symmetry, using a rigorous CC-based protocol. Several innovations allow for the first time the full and model-independent calculation of the single-particle X-ray diffraction patterns, and the resulting reconstructions fit extremely well to scanning electron microscopy (SEM) images of the particles. We also confirm experimentally the key prediction, that the CC signal-to-noise ratio is essentially independent of the average number of scatterers [17] . CC method in 2D The workflow of the CC method is illustrated schematically in Fig. 1 . The input consists of a large set of scattering images with intensities I acquired on a 2D liquid, meaning that each exposure is taken on a random ensemble of multiple identical particles. 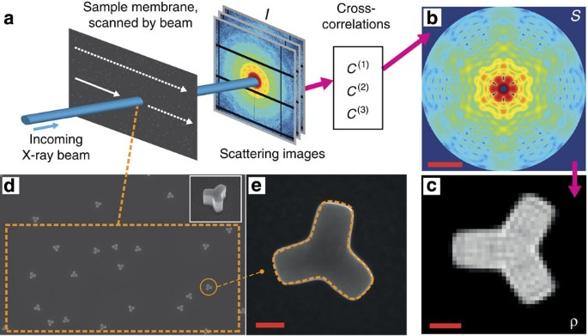Figure 1: Overview of the cross-correlation based method applied to the 2D structure determination. The flow of the protocol follows the magenta arrows: (a) the membrane carrying the gold nanostructures is scanned by the X-ray beam, and a number of scattering images, with intensitiesI, is acquired at different positions. The CCs (C(1),C(2)andC(3)) are calculated as averages over all images, and (b) the single-particle diffraction patternSis computed. The red bar represents a reciprocal space momentum transfer of 0.1 nm−1. (c) The 2D electron densityρis finally reconstructed using a phasing algorithm. The red bar corresponds to 100 nm. (d) SEM image of a small part of the sample membrane, showing the particles in random orientations. The magnification is an oblique view of a single nanostructure. The dashed orange rectangle covers an area of 14 × 6 μm2, which corresponds approximately to the X-ray beam illumination area (FWHM limit of the beam intensity in the two directions). (e) Top SEM view of a single particle, on which the dashed orange contour of the reconstructed shape is superimposed. The red bar again corresponds to 100 nm. The crucial step is the indirect determination of the diffraction pattern of a single particle in reciprocal space Figure 1: Overview of the cross-correlation based method applied to the 2D structure determination. The flow of the protocol follows the magenta arrows: ( a ) the membrane carrying the gold nanostructures is scanned by the X-ray beam, and a number of scattering images, with intensities I , is acquired at different positions. The CCs ( C (1) , C (2) and C (3) ) are calculated as averages over all images, and ( b ) the single-particle diffraction pattern S is computed. The red bar represents a reciprocal space momentum transfer of 0.1 nm −1 . ( c ) The 2D electron density ρ is finally reconstructed using a phasing algorithm. The red bar corresponds to 100 nm. ( d ) SEM image of a small part of the sample membrane, showing the particles in random orientations. The magnification is an oblique view of a single nanostructure. The dashed orange rectangle covers an area of 14 × 6 μm 2 , which corresponds approximately to the X-ray beam illumination area (FWHM limit of the beam intensity in the two directions). ( e ) Top SEM view of a single particle, on which the dashed orange contour of the reconstructed shape is superimposed. The red bar again corresponds to 100 nm. Full size image from which the 2D electron density of the particle is reconstructed, via phase retrieval, as in standard coherent diffractive imaging [18] , [19] . A polar coordinate system ( q , φ ) centred at the reciprocal space origin is the natural choice for the CC analysis. are azimuthal Fourier components, which vanish for odd n due to Friedel's law, and for which , because S is a real quantity. We define the SAXS or powder pattern as the 1-point CC, which depends only on the absolute value of the momentum transfer q . With ‹...› we denote an average over the images, and with the rotational average over the azimuthal angle ( Fig. 2a ). 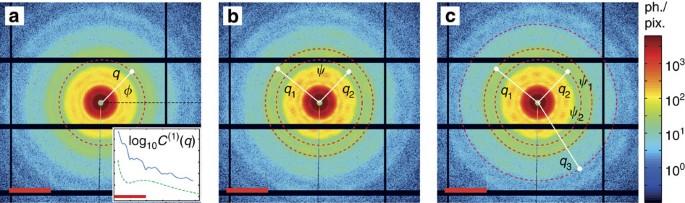Figure 2: Scattering images and cross-correlation definition. Three examples of the 3,751 different scattering images of the gold nanostructures ofFig. 1d, on a logarithmic colour scale. Superimposed are parameters pertinent (a) to the definition of the 1-point CC (equation (2)), (b) to the 2-point CC (equation (4)) and (c) to the 3-point CC (equation (6)). The red dashed circles indicate the azimuthal averages. The inset inashows the experimentalC(1)(q), whereby the green dashed curve is the subtracted background signal. The red bars correspond toq=0.1 nm−1. The 1-point CC is related to the single-particle scattering intensity by Figure 2: Scattering images and cross-correlation definition. Three examples of the 3,751 different scattering images of the gold nanostructures of Fig. 1d , on a logarithmic colour scale. Superimposed are parameters pertinent ( a ) to the definition of the 1-point CC (equation (2)), ( b ) to the 2-point CC (equation (4)) and ( c ) to the 3-point CC (equation (6)). The red dashed circles indicate the azimuthal averages. The inset in a shows the experimental C (1) ( q ), whereby the green dashed curve is the subtracted background signal. The red bars correspond to q =0.1 nm −1 . Full size image where N is the effective average number of particles in the X-ray beam, and, at this point, is simply a scaling factor. Additional structural information can be extracted from higher-order correlations. The 2-point CC results from the average of the product of two scattering intensities. It depends only on the absolute values of the two momentum transfers and the angle between them ( Fig. 2b ). The definition is [14] , [15] , [16] where δI ( q , φ )= I ( q , φ )− C (1) ( q ) is the difference of the measured intensity from its average value. The Fourier components are related to the single-particle scattering intensity by κ (2) ≤1 is a factor that depends only on the X-ray beam shape (see Methods). Equation (5) forms the basis of the CC method. Provided that the experimental data on the left-hand side are undisturbed, one can find solutions s n ( q ) that are unique to within the scaling factor and phasors exp(− iχ n ) (see Methods). In contrast to previous works [15] , [20] , to resolve these ambiguities we use the 3-point CC, which is defined in an analogous way as the 2-point CC and represents a generalization of previous suggestions [21] , [22] , and whose Fourier components yield κ (3) is an analogue of κ (2) . These equations are used to fix the values of N and χ n . Thus the remaining ambiguity in the Fourier coefficients s 0 ( q ) and { s n ( q )} n≠ 0 is eliminated, and the single-particle diffraction pattern S ( q , φ ) can be fully determined. Moreover, the number of independent equations (7) is much larger than the number of unknowns, which allows validation of the computed set of Fourier coefficients. Experimental 2D structure determinations The samples for the 2D CC demonstration experiment consisted of a large number of nominally identical 2D gold nanostructures, anchored to a membrane, with random positions and orientations ( Fig. 1d ). The membrane was scanned through a focused X-ray beam of 2 Å wavelength, and the scattering patterns were recorded with a low-noise pixel detector [23] positioned 7.2 m from the sample. We measured samples with threefold symmetric particles, with either 350 ( Fig. 1e ) or 200 nm size, and three different densities of 1.25, 10 or 40 particles per 100 μm 2 area. For each sample, 3,751 scattering images were acquired at different positions on the membrane, simulating instantaneous exposures of a 2D liquid. Such a set of images was analysed following the CC protocol, and an example of the final 2D nanoparticle structure is shown at the end of the workflow diagram in Fig. 1c , for 350 nm nanostructures and reconstructed from the data set taken on the sample with an average density of 10 particles per 100 μm 2 . Panel ( e ) of the figure demonstrates the excellent agreement of the recovered 2D shape with the shape from an SEM micrograph of an individual nanostructure. In the following, we go through the steps described in the previous section that lead to the final reconstruction, presenting the intermediate results in more detail. Figure 2 shows three examples of scattering images. The inset in ( a ) shows the 1-point CC after subtraction of the background signal taken from exposures of an empty membrane. In all three images, subtle azimuthal intensity fluctuations are visible. They are filtered out by the C (1) -azimuthal averaging, but they provide precisely the additional information that contributes to the higher-order correlations. 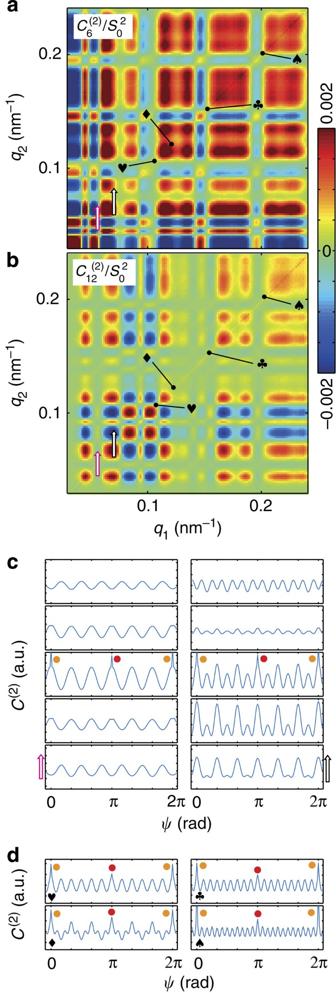Figure 3: Two-point cross-correlations. (a,b) Two-dimensional representations of the experimentally derived 2-point CC Fourier components, as a function ofq1andq2. The data are normalized withs0(q1)s0(q2), and are shown forn=6 andn=12. (c) Two-point CCsC(2)(q1,q2,ψ) as a function ofψ. The (fixed)q1and (variable)q2values follow the paths of the magenta arrows ina,bfor the plots in the left column, and of the black arrows ina,bfor those in the right column. The spikes observed forq1=q2atψ=0, owing to noise and interparticle interference, and atψ=π, owing only to interparticle interference, are marked with orange and red dots, respectively. (d) Diagonal 2-point CCC(2)(q1,q2,ψ), as a function ofψ, for differentqvalues corresponding to the differently labelled black dots on the diagonal ina,b. The spikes are marked as described inc. Figure 3 is devoted to the 2-point CCs. Panels ( c ) and ( d ) show examples of C (2) ( q 1 , q 2 , ψ ), while panels ( a ) and ( b ) display the coefficients and , respectively, where the 2D representation as a function of q 1 and q 2 serves to emphasize the importance of the non-diagonal ( q 1 ≠ q 2 ) CCs in our protocol. The encoded information was then used, in combination with that from the 3-point CC, to extract the Fourier components { s n ( q )} n ≠0 of the single-particle diffraction intensity. In the analysed range of transferred momentum (0.009≤ q ≤0.24 nm −1 ), only the coefficients with n =6, 12, 18, 24, 30, displayed in Fig. 4a , could be calculated consistently and validated. 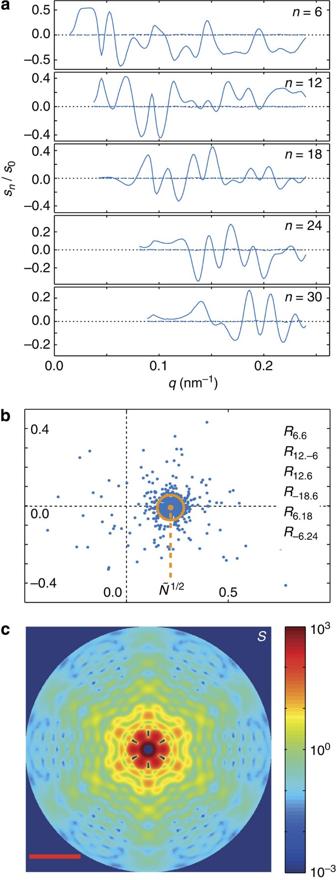Figure 4: Single-particle diffraction pattern. (a) Fourier coefficientsn(q) of the single-particle diffraction pattern, extracted from the experimental CCs, as a function ofq. The data are shown forn=6, 12, 18, 24, 30, and are rescaled withs0(q). The continuous and dashed curves correspond to the real and imaginary parts, respectively. (b) Complex plane representations of the ratiosRnm(qa,qb,qc) (equation (13)), for differentnandmmultiples of 6, for fixedqa=0.066 nm−1andqb=0.115 nm−1, and for a large number ofqc. The centroid point in orange is the median of all points, and the orange circle encloses the area containing the closest 80% of all points. The imaginary part of the centroid point is negligible, and its real part corresponds to, with. (c) Single-particle diffraction patternS(q,φ), on a logarithmic colour scale, and defined over a disk-shaped region with maximal reciprocal-space frequencyqmax=0.24 nm−1. The dark regions in the corners are deficient of data. The red bar corresponds toq=0.1 nm−1. Figure 4b displays ratios of 3-point CC components to the single-particle coefficients s n , as points in the complex plane (see equation (13) in the Methods for a precise formulation) and validity is inferred by the fact that almost all such points fall at the same real-positive value, which is proportional to . This determines the effective average number of scattering particles to be N ≈20. Other coefficients were not considered further, because they could neither be determined self-consistently nor validated (see Supplementary Figs S1 and S2b–e ). Their contribution is in any case negligible ( Supplementary Fig. S2a ), with the exception of n =2, and the motivations for considering s 2 ( q ) as an artifact are described in detail in the Supplementary Methods . Figure 3: Two-point cross-correlations. ( a , b ) Two-dimensional representations of the experimentally derived 2-point CC Fourier components , as a function of q 1 and q 2 . The data are normalized with s 0 ( q 1 ) s 0 ( q 2 ), and are shown for n =6 and n =12. ( c ) Two-point CCs C (2) ( q 1 , q 2, ψ ) as a function of ψ . The (fixed) q 1 and (variable) q 2 values follow the paths of the magenta arrows in a , b for the plots in the left column, and of the black arrows in a , b for those in the right column. The spikes observed for q 1 = q 2 at ψ =0, owing to noise and interparticle interference, and at ψ = π , owing only to interparticle interference, are marked with orange and red dots, respectively. ( d ) Diagonal 2-point CC C (2) ( q 1 , q 2, ψ ), as a function of ψ , for different q values corresponding to the differently labelled black dots on the diagonal in a , b . The spikes are marked as described in c . Full size image Figure 4: Single-particle diffraction pattern. ( a ) Fourier coefficient s n ( q ) of the single-particle diffraction pattern, extracted from the experimental CCs, as a function of q . The data are shown for n =6, 12, 18, 24, 30, and are rescaled with s 0 ( q ). The continuous and dashed curves correspond to the real and imaginary parts, respectively. ( b ) Complex plane representations of the ratios R nm ( q a , q b , q c ) (equation (13)), for different n and m multiples of 6, for fixed q a =0.066 nm −1 and q b =0.115 nm −1 , and for a large number of q c . The centroid point in orange is the median of all points, and the orange circle encloses the area containing the closest 80% of all points. The imaginary part of the centroid point is negligible, and its real part corresponds to , with . ( c ) Single-particle diffraction pattern S ( q , φ ), on a logarithmic colour scale, and defined over a disk-shaped region with maximal reciprocal-space frequency q max =0.24 nm −1 . The dark regions in the corners are deficient of data. The red bar corresponds to q =0.1 nm −1 . Full size image The single-particle diffraction intensity S ( q , φ ), shown in Fig. 4c , is obtained by merging the valid coefficients {s n ( q )} n = 6,12,18,24,30 together with s 0 ( q ), and obviously shows sixfold symmetry. Results from simulations suggest that the small regions with negative intensity are owing to non-perfectly identical scatterers (see Supplementary Fig. S3 ). S was subsequently used as input to a phase retrieval algorithm for reconstructing the 2D electron density ρ , shown in Fig. 5a , normalized to be on average unity in the interior of the structure. We estimate the spatial resolution to be ~17.5 nm from the average sharpness of the edge of the structure, defined as the mean separation between the 0.1 and 0.9 contour levels. The high reliability of the phase retrieval reconstruction was assessed from the phase retrieval transfer function (PRTF) [24] , shown as a function of the momentum transfer q in Fig. 5b , whose value is well above 0.5 in the relevant range in reciprocal space ( q <0.18 nm −1 ). 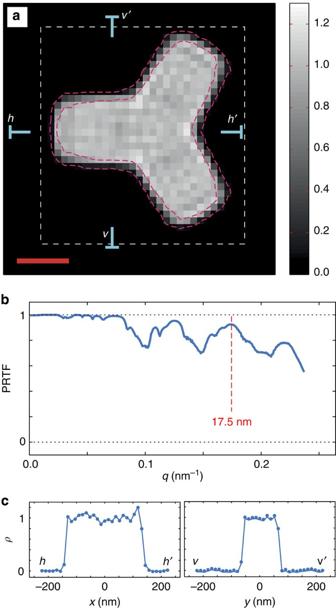Figure 5: Two-dimensional structure. (a) Averaged 2D electron densityρfrom 50 reconstructions.ρis normalized to be on average unity in the core of the structure. One real-space pixel corresponds to 13.0 nm, and the red bar corresponds to 100 nm. The dashed white rectangle delimits the region of compact support imposed during the iterative phase retrieval procedure. The two dashed magenta lines are theρ=0.9 andρ=0.1 contour levels, and their average separation provides an estimate of the achieved resolution of 17.5 nm. (b) Phase-retrieval transfer function PRTF(q) resulting from the 50 reconstructions, as a function ofq. The red dashed vertical line marks theqvalue corresponding to the resolution estimated ina. (c) Horizontal section (h–h′) and vertical section (v–v′) through the 2D electron densityρ, at the positions marked in cyan ina. Figure 5: Two-dimensional structure. ( a ) Averaged 2D electron density ρ from 50 reconstructions. ρ is normalized to be on average unity in the core of the structure. One real-space pixel corresponds to 13.0 nm, and the red bar corresponds to 100 nm. The dashed white rectangle delimits the region of compact support imposed during the iterative phase retrieval procedure. The two dashed magenta lines are the ρ =0.9 and ρ =0.1 contour levels, and their average separation provides an estimate of the achieved resolution of 17.5 nm. ( b ) Phase-retrieval transfer function PRTF( q ) resulting from the 50 reconstructions, as a function of q . The red dashed vertical line marks the q value corresponding to the resolution estimated in a . ( c ) Horizontal section (h–h′) and vertical section (v–v′) through the 2D electron density ρ , at the positions marked in cyan in a . Full size image For the smaller 200 nm particles, we obtained similar results, illustrated in Fig. 6 . In this case, the resolution is estimated to be ~13.5 nm (corresponding to q =0.23 nm −1 ). For both 350 and 200 nm particle sizes, the experimental data measured at the three different surface densities imply average numbers of scattering particles of N ≈2.5/20/80, which are consistent with the known sample densities, beam size and beam shape (see Methods). Moreover, as can be seen in Fig. 7a , the data taken on the different samples demonstrate that the 2-point CCs scale properly with N , as required by equation (5), with some deviations at larger q . Equivalently, Fig. 7b show that the extracted s 0 ( q ) and s n ( q ) are in general independent of N . Only at large q is there a noticeable suppression of s n with decreasing N , an observation that we cannot explain at present. 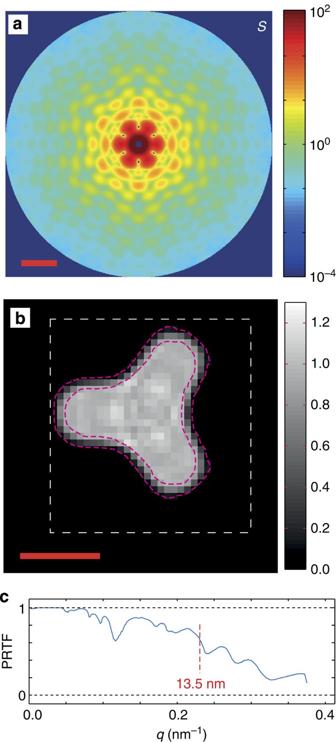Figure 6: Results with 200 nm particles. (a) Single-particle diffraction patternS(q,φ). The presentation is the same as inFig. 4c, with maximal reciprocal-space frequencyqmax=0.37 nm−1. The red bar corresponds toq=0.1 nm−1. (b) Averaged 2D electron densityρfrom 50 reconstructions. The presentation is the same as inFig. 5a, with one pixel corresponding to 8.4 nm, and the red bar to 100 nm. The resolution, given by the distance of the two magenta contours, is 13.5 nm. (c) Phase-retrieval transfer function PRTF(q) resulting from the 50 reconstructions, as a function ofq. The red dashed vertical line marks theqvalue corresponding to the resolution estimated inb. Figure 6: Results with 200 nm particles. ( a ) Single-particle diffraction pattern S ( q , φ ). The presentation is the same as in Fig. 4c , with maximal reciprocal-space frequency q max =0.37 nm −1 . The red bar corresponds to q =0.1 nm −1 . ( b ) Averaged 2D electron density ρ from 50 reconstructions. The presentation is the same as in Fig. 5a , with one pixel corresponding to 8.4 nm, and the red bar to 100 nm. The resolution, given by the distance of the two magenta contours, is 13.5 nm. ( c ) Phase-retrieval transfer function PRTF( q ) resulting from the 50 reconstructions, as a function of q . The red dashed vertical line marks the q value corresponding to the resolution estimated in b . Full size image Figure 7: Dependence on particle size and surface density. Data for the 350 nm nanoparticles (left column) and 200 nm particles (right column), and for three different particle surface densities corresponding to N =2.5 (red), N =20 (blue) and N =80 (black). ( a ) Examples of diagonal 2-point CCs C (2) ( q 1 , q 2, ψ ), as a function of ψ , for two different q values for each particle size. The data are rescaled with N . ( b ) Zeroth-order Fourier coefficients s 0 ( q ) of the single-particle diffraction pattern, as a function of q . The background signal is represented by the dashed green curve. ( c ) Amplitude of the Fourier coefficients s n ( q ) of the single-particle diffraction pattern, as a function of q . The values are shown for n =6 and n =12 and are rescaled with s 0 ( q ) calculated from the N =20 data set. ( d ) Average deviations Δ s 6 ( q ) of the Fourier coefficients s 6 ( q ), as a function of q (Methods). Full size image In the framework of X-ray diffraction, the results obtained represent the first model-independent experimental proof-of-principle of the CC method applied to 2D structure determination. From the low single-particle signal-to-background ratio highlighted in Fig. 7b , it is manifest that standard 2D structure determination by phase retrieval from a unique single-particle diffraction image would be unsuccessful. The difference between the reconstructed shape and the real shape of one representative particle is much smaller than the achieved resolution of ~15 nm, which is not an intrinsic limitation of the method, but rather reflects the difficulty of fabricating identical but randomly oriented nanostructures. Characteristic features of the protocol, described in detail in the Methods, are the ‘diagonalization’ procedure to consistently solve the 2-point equation (5), and the use of the 3-point equation (7) for validation of the single-particle diffraction Fourier components. In this way, the single-particle diffraction pattern is determined unambiguously and in a model-independent fashion. This distinguishes our protocol from previous work. Saldin et al . [16] derived the phases of such Fourier components from previous knowledge of the elongated shape of the particles under investigation and did not explicitly discuss how the overall ratio between s 0 and { s n } n >0 was determined. We found this ratio to be decisive for the quality of the reconstructed 2D structures. As s 0 and { s n } n >0 scale as 1/ N and , respectively (equations (3) and (7)), underestimating the average number of scatterers N or setting κ (2) =1, as for a flat-top beam profile, results in a decrease of contrast in the calculated single-particle diffraction pattern. Using such reduced contrast images as input for the phasing algorithm, we were able to produce prominent, ball-shaped artefacts, of the sort present in the final reconstruction presented in ref. 16 . The basic equations (5) and (7) are strictly valid in the limit of an infinite number of scattering images, N im , which is necessary for averaging out the contributions to the CCs arising from pairs of particles in the same image ( Supplementary Note 1 ). In practice, this means that a ‘sufficient’ number of images has to be acquired, which leads one to consider the fluctuations, or signal-to-noise, of the CC at large N im and as a function of the number of scatterers N . The signal-to-noise of the 2-point CC was evaluated analytically for the 3D case [17] , and found to be independent of N , unless the background scattering is comparable to that from an individual particle, in which case increasing N becomes advantageous. These findings are supported by an appropriate analysis of our data. We take the coefficients { s n ( q )} n >0 to be the signal, which is N -independent, hence estimating the signal-to-noise Δ s n ( q ) becomes equivalent to estimating the noise. Figure 7d displays Δ s n ( q ) derived from the experimental data for N im =100 (Methods), and for three different N =2.5, 20 and 80. For the 350 nm particles, Δ s n ( q ) is found to be independent of N , while for the case of the smaller, 200-nm-sized structures, which have a less favourable signal-to-background scattering ratio ( Fig. 7b ), a decrease in Δ s n ( q ) at large q is evident as N is increased from 2.5 to 20. A multiparticle diffraction image is the sum of the images of each particle plus an interference term from each pair of particles, if these are closer to one another than the transverse coherence length. As this term is phase-modulated by the interparticle distance, random particle positions cause its contribution to C (2) ( q 1 , q 2 , ψ ) to average out in the limit of an infinite number of images, with the exception at q 1 = q 2 and ψ =0 or ψ = π (see Supplementary Note 2 ). This explains the two spikes of the same height present in the diagonal CCs, which are proportional to the square of the average number of particles in a coherence area and which are marked with orange and red dots in Figs 3d and 7a . The optimal size of the coherence area is thus twice the size of a single particle, in order to achieve Nyquist sampling and at the same time to minimize the number of interfering particles. It is worth mentioning the other factors that modify the CC identities. Poisson noise and (uncorrelated) background scattering result in a spike at ψ =0 in C (2) ( q 1 , q 2 , ψ ) for q 1 = q 2 ( Supplementary Fig. S4 and Supplementary Note 3 ), marked with orange dots in Figs 3d and 7a . Because perturbations from noise and interference effects both appear as localized spikes, it is not difficult to evaluate their importance, and in our case we could also easily verify that they were filtered out during the procedure to obtain the coefficients s n (Methods). A preferred orientation of the identical particles also requires corrections of (5) and (7) ( Supplementary Note 1 ). Finally, a brief discussion should be made of the general case of non-identical scattering particles. If the situation can be reduced to a finite number of 2D particle species with uncorrelated orientation, the validity of equation (5) is restored by replacing the right-hand side with a sum over the species , and a similar modification is necessary in (3) and (7). This opens the door to studying systems of different 2D particle species in ‘chemical equilibrium’, or of identical 3D particles presenting a finite number of different 2D projections with respect to the incoming beam. For the simplest case of a two-component particle/solvent system, the separately measured contribution to the CCs of the solvent alone can be subtracted. In our experiments, the solvent is represented by the membrane on which the nanoparticles were anchored, and thus we determined solvent contributions using the scattering data from an empty membrane. The clear contribution to the 1-point CC, which we attribute to membrane thickness fluctuations, was taken into account by background subtraction (inset of Fig. 2a ). For the 2- and 3-point CCs, however, we infer an effectively vanishing contribution. There is a number of 2D static systems that are not strictly included in the framework described above, and which are studied or characterized by SAXS measurements at synchrotron sources. Evaluating the higher-order CCs of the scattered images is trivial, and could already at present disclose additional information [25] , [26] , for example the average anisotropy of the domains in magnetic storage media or of the pores in fuel cell membranes. The CC analysis may also be useful to access short-range structural properties in disordered, slowly changing systems. Wochner et al . [27] have used the diagonal 2-point CC, derived from synchrotron X-ray coherent diffraction data from highly concentrated suspensions of PMMA nanospheres, to identify the preferential symmetry of 3D clusters [25] that form temporarily within the sample. Regarding possible future investigations on 3D structural features of macromolecules or other particles in solution, which exploit the brilliance of XFEL radiation sources, it appears that applying the CC method in the spirit of its original formulation [13] is a suitable approach; dynamical information may be accessed through the straightforward generalization of the CC analysis to laser pump/X-ray probe scattering images, or even to scattering data obtained with X-ray split-and-delay data [28] , [29] . The present 2D demonstration experiment and its discussion have direct relevance to the 3D case, regarding the effects of interparticle interference and of the unavoidably non-uniform beam intensity profile, as well as the independence of the signal-to-noise from the average number of scattering particles. Increasing the dimensionality from 2D to 3D, however, calls for some additional considerations. The 3D single-particle diffraction pattern can be decomposed into spherical harmonics and there are clearly more components than for the 2D case. In contrast, the number of 2-point CC identities [13] , [30] in 3D is the same as in 2D: Here, are the components of C (2) ( q 1, q 2, ψ ) with respect to the n -th order Legendre polynomials in cos ψ . Elser [31] has recently shown that without additional assumptions, these equations cannot be solved for the coefficients s nm ( q ) to the same extent as in 2D (that is, to within the parameters N and χ n ). These assumptions may include a priori knowledge of the particle symmetries, which reduce the number of independent parameters in S ( q , θ , φ ). For axially symmetric particles, only the s n 0 coefficients are non-vanishing [13] . Similarly, if the particles exhibit icosahedral symmetry, as is often the case in viruses [21] , for each n there is at most one component proportional to an icosahedral harmonic [32] . In both cases, the problem becomes equivalent to the 2D case. In general, equation (9) may be interpreted as constraints on S , to be used in addition to the 3D equivalent of (3): for modelling a 3D electron density of the particles at higher resolution than is possible with equation (10) alone. Regarding the use of the 3-point CC, the definition (6) is applicable also in the 3D case. It represents a generalization of that put forward in ref. 21 , in that it implies access to three instead of two reciprocal space vectors. Although the experimental geometry in X-ray diffraction experiments limits these triples to be coplanar, the new definition provides additional constraints that can be exploited for fixing the s nm ( q ) coefficients, in a similar manner to that described in ref. 21 . At large scattering angles, straightforward corrections are necessary for the anisotropic scattering owing to linear polarization [33] of the incoming beam and for the curvature of the Ewald sphere. However, the bottleneck to achieving subnanometer resolution is that the key parameter determining the precision of the CC method is the number of scattered photons per coherent pixel and per particle [17] , which especially for macromolecules may be well below unity. There is no doubt that the method, as any other single-particle approach, would greatly profit from increases in the X-ray beam fluence. The adavantage of using CCs is that the low scattering power can be compensated simply by drastically increasing the number of acquired images, although even weak solvent scattering may become a significant, additional issue. For this reason, the next round of experiments, which will attempt to identify nm-scale features of 3D molecules in liquid or aerosol jets, is considered crucial for the development of the CC method. Samples The samples were prepared on a 2 × 2 mm 2 Si 3 N 4 membrane of 200 nm thickness, held by a Si wafer and coated with a Cr/Au (5/20 nm) seed layer. The gold nanoparticles were fabricated by electroplating into a 500-nm-thick PMMA resist mould, patterned by electron beam lithography. More details on the nanofabrication procedures can be found elsewhere [34] . The particles with designed threefold symmetry were randomly oriented about the axis perpendicular to the membrane, and placed in random positions within an 800 × 800 μm 2 field, with the restriction of a 500 nm minimum interparticle distance. The measurements were performed on several samples, which differed in the diameter/thickness of the nanostructures (350/350 nm, respectively, 200/250 nm), and in the average particle surface density (1.25/10/40 particles per 100 μm 2 area). Beamline setup and data acquisition The X-ray measurements were performed at the cSAXS beamline (X12SA) of the Swiss Light Source synchrotron at the Paul Scherrer Institute. The beamline was set to a photon energy of 6.2 keV, with a relative bandwidth of ~10 −4 obtained with a Si(111) double-crystal monochromator, and with a flux of ~2·10 11 photons per second. The beam was focused onto the sample; the horizontal and vertical focusing were achieved by bending appropriately the second monochromator crystal and the higher-harmonic rejection mirror, located 5.5 and 4.5 m upstream of the sample, respectively. The beam size was 14 × 6 μm 2 FWHM (see below), and the transverse coherence length was at least twice the dimension of a nanostructure, that is, at least 700 nm. The scattered X-rays were transported through an evacuated flight tube to the detector, which was placed 7.2 m behind the sample. The detector [23] was a Pilatus 2M, with 1675 × 1475 square pixels of 172 μm size, and was protected from the direct beam by a central beamstop. The X-ray beam diameter at the detector position, measured with an attenuated beam and without inserted sample, corresponded to 3–4 detector pixels. For each sample, 3,751 scattering images of 1 s acquisition time were taken, scanning the membrane on a 121 × 31 point rectangular grid, which covered an area of 600 × 600 μm 2 . X-ray beam shape parameters and beam shape assessement The correction parameters κ (2) and κ (3) and the relation between the effective parameter N and the particle density are determined by the 2D intensity illumination function at the sample, Ω( x , y ), according to κ ( j ) =( ∬ d x d y Ω j )/( ∬ d x d y Ω) ( Supplementary Note 4 ). Ω( x , y ) was determined experimentally as described in Supplementary Fig. S5 and the Supplementary Methods , and resulted in κ (2) ≈0.26, κ (3) ≈0.14 and N / N FWHM ≈π 2 /4, where N FWHM is the number of particles in the FWHM area of the beam. Discretization of the diffracted intensity The position of the scattering centre on the pixel detector was established by averaging a number of centre-of-gravity points of pairs of opposite Bragg reflections produced by a 2D hexagonal periodic array ( Supplementary Fig. S5c ). A polar ‘spider-web’ grid was defined around this centre as ( q a, φ k ), with a {1,…, N q } and φ k = k 2 π k/N φ , for k {0,…, N φ −1}, which also prescribes the binning of the detector pixels. The scattering intensities in polar coordinates I ( q a , φ k ) were then calculated as the average over the pixels belonging to the same polar bin. For the 350-nm-sized structures, q a was defined to be spaced by the equivalent of two detector pixels (0.0015, nm −1 ), and three different q a ranges were considered: 0.009–0.006 nm −1 ( N q =35), 0.015–0.12 nm −1 ( N q =71) and 0.03–0.24 nm −1 ( N q =141), with N φ =32, 64 and 128 azimuthal sectors, respectively. For the 200 nm structures, q a was defined to be spaced by the equivalent of four detector pixels (0.003 nm −1 ), and four different q a ranges were considered: 0.009–0.06 nm −1 ( N q =18), 0.015–0.12 nm −1 ( N q =36), 0.03–0.24 nm −1 ( N q =71) and 0.06–0.37 nm −1 ( N q =106), with N φ =32, 64, 128 and 256 azimuthal sectors, respectively. Computation of the single-particle diffraction pattern: theory The core of the presented work concerns the calculation of the single-particle diffraction pattern S ( q , φ ) from the CCs, that is, the solution of equations (3), (5) and (7) for s n ( q ). Let q a be a finite, discrete set of q values. Inspired by Kam and coworkers [22] , and also by Saldin and coworkers [30] , for n ≠0 we use the 2-point CC coefficients to define the Hermitian matrix , which can be diagonalized to yield real eigenvalues λ n,i ( i {1,…, N q }). We designate λ n, 1 to be the largest positive eigenvalue and write the eigenvector decomposition as with and ( i {2,…, N q }). Note that the vector s n is defined to within an overall phase χ n . According to (5), one expects a single non-vanishing, positive eigenvalue λ n ,1 . Therefore, a signature of the various perturbations, such as finite number of images, shot noise, uncorrelated background noise, interparticle interference, preferred particle orientation and inequivalent particles, being small is that which is equivalent to requiring the second term on the right-hand side of (11) to be negligible. If this is the case, one uses the eigenvectors s n to compute the ratios The last equality arises from the 3-point CC equation (7) in combination with equation (15) below, and enables fixing χ n and the effective number of particles N . These parameters are actually overdetermined, which allows for an additional validation. Finally, the desired single-particle diffraction components are set to and Computation of the single-particle diffraction pattern: practice The 2D reciprocal space discretization described above was used for all calculations, whereby each relevant equation translates in a straightforward way to the discretized form. Before the computation of the CC, the average intensity was subtracted from each individual diffraction image, in order to eliminate eventual beamline artefacts that result in configuration-independent contributions to the scattering intensity. Diagonalization along the lines of equation (11) was performed for even n in the three or four q a ranges for 350 or 200 nm structures, respectively ( Supplementary Methods ). Requirement (12) was translated into , and, if not fulfilled, the lower limit of the q a range was raised (due to the high sensitivity to disturbances of C n,ab , when s n ≈0 at low q a ). The s n from the q a ranges were then merged by matching their phase at overlapping q a intervals. The phase relations of equation (13), for the relevant n and m and for a number of different q a , q b and q c , represent an overconstrained system of first-order equations in the overall correction phases χ n , which is straightforwardly solved following the procedure described in the Supplementary Methods . Because of the mirror symmetry of the nanostructures considered in the experiments, the s n can be chosen real, so that the phase ambiguity is effectively only a sign ambiguity. However, the method to fix the overall phases of the s n is absolutely general, as demonstrated in Supplementary Fig. 6 . Finally, the parameter N was chosen to best fulfill the amplitude relation of (13), for various n , m . The final values of s 0 ( q a ) and s n ( q a ) were then determined using (14) and (15), and the coefficients with n 6 N were used to calculate the single-particle diffraction pattern S ( q , φ ) with equation (1) on a polar grid with N φ =128 azimuthal points for the 350 nm structures (| n |≤30) and N φ =256 for the 200 nm structures (| n |≤48). Phase retrieval For reconstruction of the structures, the polar expressions for single-particle diffraction intensities S ( q , φ ) were interpolated onto a Cartesian grid ( q x , q y ), suitable for fast Fourier transform algorithms. For the 350 nm particles, the grid was 512 × 512 points with q max =0.24 nm −1 , which corresponds to a real-space pixel size of 13.0 nm. For the 200 nm structures, the grid was 500 × 500 points with q max =0.37 nm −1 , giving a real-space pixel size of 8.4 nm. A high-pass version of the structure autocorrelation [35] , given by the inverse Fourier transform of S ( q x , q y ), was used to determine the size of the autocorrelation support. The support region of the 2D electron density was then defined as a rectangle of half that size, enlarged by one pixel in each direction to avoid artificial sharpening of the reconstruction edges. The reconstruction of the 2D structures was performed with an iterative transform algorithm using the above-mentioned support as real-space constraint and as reciprocal space modulus constraint. The procedure [36] consisted of a series of 45 hybrid input–output [37] iterations followed by five error-reduction steps, repeated until a total of 1,000 iterations was reached. In the reciprocal space projection steps, the algorithm was allowed to fill the regions obscured by the beamstop ( q <0.009 nm −1 ) and those with negative S ( q x , q y ) values. As the polar reconstruction of S ( q , φ ) is limited to a disk-shaped region, the Cartesian representation has large regions of missing data at the corners. To avoid artifacts from the abrupt interruption of data at the boundary of this disk, we used Fourier-weighted projections [36] with a non-binary mask, suitable to allow the algorithm to slightly extrapolate the measured data by a few pixels without introducing a large number of free parameters in the reconstruction. Starting with different random phase sets, 50 reconstructions were performed, which were then registered within a small fraction of a pixel [38] , and averaged to obtain the final 2D structure shown in Fig. 5a . The reliability of the reconstruction was evaluated from the azimuthal average of the PRTF [24] , calculated from the 50 reconstructions. Signal-to-noise estimates For a given number of scattering images, N im , we estimate the noise Δ s n ( q ) of the Fourier coefficients of the single-particle diffraction pattern as follows: Here, N sets is the number of sets of scattering images used for the estimate, each consisting of N im randomly chosen images from the full set of 3,751. s σ,n is the coefficient calculated from the images in the set σ , and s ref, n is the reference value, calculated from all 3,751 images. How to cite this article: Pedrini, B. et al . Two-dimensional structure from random multiparticle X-ray scattering images using cross-correlations. Nat. Commun. 4:1647 doi: 10.1038/ncomms2622 (2012).